Disruption of astrocyte–vascular coupling and the blood–brain barrier by invading glioma cells Astrocytic endfeet cover the entire cerebral vasculature and serve as exchange sites for ions, metabolites and energy substrates from the blood to the brain. They maintain endothelial tight junctions that form the blood–brain barrier (BBB) and release vasoactive molecules that regulate vascular tone. Malignant gliomas are highly invasive tumours that use the perivascular space for invasion and co-opt existing vessels as satellite tumour form. Here we use a clinically relevant mouse model of glioma and find that glioma cells, as they populate the perivascular space of preexisting vessels, displace astrocytic endfeet from endothelial or vascular smooth muscle cells. This causes a focal breach in the BBB. Furthermore, astrocyte-mediated gliovascular coupling is lost, and glioma cells seize control over the regulation of vascular tone through Ca 2+ -dependent release of K + . These findings have important clinical implications regarding blood flow in the tumour-associated brain and the ability to locally deliver chemotherapeutic drugs in disease. It is now well established that astrocytes play important roles in supporting normal brain function [1] . This is largely accomplished by astrocytic processes that form endfeet covering ~99% of the cerebrovascular surface [2] . Astrocyte endfeet, in conjunction with pericytes [3] , help to maintain the expression of endothelial tight junction proteins, transporters and enzymes, which together comprise the BBB [4] , [5] , [6] . In addition, astrocytes can release a number of vasoactive molecules from their endfeet onto the underlying vascular smooth muscle cells (VSMCs), regulating vascular tone [7] . This process, called functional hyperaemia or neurovascular coupling (NVC), adjusts local cerebral blood flow to match regional neuronal energy demand. NVC is accomplished by translating neuronal activity into increases in astrocytic [Ca 2+ ] i , which causes the generation and/or release of several vasoactive molecules including the arachidonic acid (AA) metabolites epoxyeicosatrienoic acids, prostaglandin E 2 (PGE 2 ) and 20-HETE or K + . These metabolites act on smooth muscle cells lining cerebral arterioles causing them to dilate or constrict [7] , [8] , [9] , [10] , [11] . Primary glial-derived brain tumours, gliomas, are highly invasive cancers, which often migrate along existing brain structures including white matter tracks and blood vessels [12] , [13] . Endothelial-derived bradykinin initially attracts glioma cells to the vasculature [14] and the extracellular matrix surrounding these blood vessels is enriched with molecules, such as fibronectin and vitronectin, that promote cell migration [15] . Interactions of glioma cells with the vasculature occurs in three distinct ways: (1) perivascular invasion of migrating glioma cells along the preexisting vasculature and (2) co-option of preexisting host vessels [16] during initial tumour growth or by small satellite tumours. As the disease progresses and the tumour mass grows, co-opted vessels eventually undergo apoptosis and (3) angiogenesis is induced by the release of angiogenic molecules such as vascular endothelial growth factor (VEGF) [17] at the fringe of the tumour mass. In this study, we exclusively focused on the interaction of migrating glioma cells with the preexisting vasculature outside of the main tumour mass. Given the extensive coverage of cerebral vessels by astrocytic endfeet [2] , we asked whether gliomas invading along or co-opting vessels might alter astrocyte–vascular interactions at the preexisting vasculature. Using several clinically relevant mouse models of glioma, we show that a vast majority of human glioma cells that travelled outside of the main mass associate with blood vessels and insert themselves between the endfeet and the endothelial wall of the preexisting blood vessel, confirming previous reports using rodent glioma cell lines [13] , [18] , [19] . The loss of contact between endfeet and blood vessels leads to a loss of tight junctions (TJs) thereby causing a focal breach of the BBB allowing blood-borne molecules to enter the brain parenchyma even far away from the main tumour mass. Furthermore, the physical dislocation of astrocytes from the blood vessels and subsequent encasing of vessels by gliomas disrupts astrocyte–vascular coupling. Importantly, single glioma cells are sufficient to locally open the BBB and focally disrupt gliovascular coupling. These findings have important clinical implications regarding blood flow in the tumour-associated brain and the ability to locally deliver chemotherapeutic drugs in disease. Glioma cells associate with blood vessels Gliomas interact with both existing and newly generated blood vessels at different stages of the disease. Early on, existing vessels serve as a pathway for tumour invasion [20] . Later, new vessels generated through angiogenesis [21] , supply blood-borne nutrients to support tumour growth. This period is preceded by vascular co-option where gliomas form cuff-like clusters around resident vessels [18] . Perivascular invasion and vascular co-option continue throughout the disease as tumour cells spread and create satellite tumours. The principle objective of this study was to study the interaction of gliomas with the existing vasculature. To do so, we used mouse models of glioma that replicate salient features of the disease including perivascular invasion [20] , vascular co-option [16] , [18] and angiogenesis [17] . As a first step, we investigated the extent to which glioma cells associate with blood vessels, paying specific attention to vessel type and size. To visualize tumour cells in brain, we implanted eGFP-expressing human glioma cells ( D54-eGFP ) into the cortex of immunodeficient scid mice and allowed cells to proliferate and invade for 2–4 weeks. Almost all D54 glioma cells, outside of the main tumour mass, associate with CD31 (PECAM-1)-labelled blood vessels ( Fig. 1a ). To assure that this phenomenon is a general property of glioma cells, we generated gliomas using four additional glioma sources; one mouse-derived glioma cell line ( Gl261-dsRed ) and three different patient-derived glioma xenolines ( GBM22 , GBM39 and GBM14 ). The latter tissue has been exclusively propagated in the flanks of nude mice to preserve protein expression of the original tumour [22] . As with D54 glioma cells, the mouse- and patient-derived tumour cells that migrated into the parenchyma were frequently associated with blood vessels ( Fig. 1b,c ; Supplementary Fig. 1 ). For further studies, we focused on D54-eGFP cells, as well as GBM22 (classified as mesenchymal subtype) and GBM14 (classified as classical subtype). Similarly to D54 gliomas, GBM22 gliomas form loose tumour borders with cells invading chain-like into the parenchyma using blood vessels as a scaffold ( Fig. 1b ; Supplementary Fig. 1e,f ). In each preparation, the vast majority of cells contact a vascular surface ( Fig. 1d–f ). 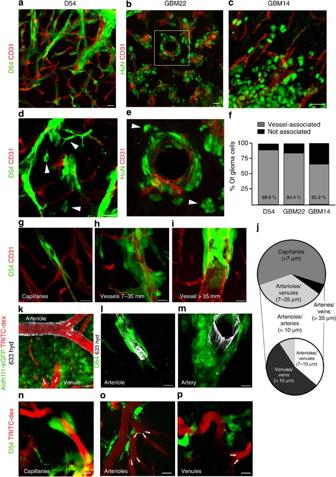Figure 1: Glioma cells can associate with blood vessels of all sizes and types. Immunofluorescence of CD31 (PECAM) and eGFP-expressing human glioma cells (D54) (a) or patient-derived xenograft linesGBM22(b) andGBM14(c) implanted in the cerebrum of immunodeficient mice highlighting the high number of invading glioma cells found along the vasculature. To be scored ‘vessel associated’, we required overlap of pixels of the endothelial cell (red) and the tumour cell (green) label in 1–2 μm single planes of confocal images. Only a minority of cells is not found along the vasculature (d–f, arrow heads). Perivascular glioma cells can associate with capillaries (<7 μm) (g), penetrating arterioles or venules (7–35 μm) (h) and large arteries or veins (>35 μm) (i). Quantitative analysis based on 1,634 cells in five random sections from each slice and three slices from four different animals (j). Immunofluorescence of Alexa Fluor 633 hydrazide dye (633 hyd, white) and eGFP-expressing astrocytes (Aldh1l1-eGFP) or human glioma cells (D54) implanted in the cerebrum of immunodeficient mice allowing to distinguish arterioles/arteries from venules/veins and capillaries (k–m). Black font was used to describe white labels in confocal images. Quantification of 75 sections from four tumour-bearing animals show that glioma cells associate with every type of vessel (j).In vivovisualization of eGFP-expressing human glioma cells implanted in the cerebrum of immunodeficient mice found invading along the vasculature outlined by tetramethylrhodamine-dextran (TRITC-dex). Arterioles show divergent and venules show convergent blood flow at branch points (arrows ink,o,p). Perivascular glioma cells can associate with capillaries (n), penetrating arterioles (o), penetrating venules (p). Scale bar, 20 μm. Statistical data: (a,d)n=4 animals; (b)n=5 animals; (c)n=7 animals; (f) quantification forn=4 D54 animals,n=3 GBM22 and GBM14 animals; (g–m)n=9 animals; (n–p)n=34 animals. Figure 1: Glioma cells can associate with blood vessels of all sizes and types. Immunofluorescence of CD31 (PECAM) and eGFP-expressing human glioma cells ( D54 ) ( a ) or patient-derived xenograft lines GBM22 ( b ) and GBM14 ( c ) implanted in the cerebrum of immunodeficient mice highlighting the high number of invading glioma cells found along the vasculature. To be scored ‘vessel associated’, we required overlap of pixels of the endothelial cell (red) and the tumour cell (green) label in 1–2 μm single planes of confocal images. Only a minority of cells is not found along the vasculature ( d – f , arrow heads). Perivascular glioma cells can associate with capillaries (<7 μm) ( g ), penetrating arterioles or venules (7–35 μm) ( h ) and large arteries or veins (>35 μm) ( i ). Quantitative analysis based on 1,634 cells in five random sections from each slice and three slices from four different animals ( j ). Immunofluorescence of Alexa Fluor 633 hydrazide dye (633 hyd, white) and eGFP-expressing astrocytes ( Aldh1l1-eGFP ) or human glioma cells ( D54 ) implanted in the cerebrum of immunodeficient mice allowing to distinguish arterioles/arteries from venules/veins and capillaries ( k – m ). Black font was used to describe white labels in confocal images. Quantification of 75 sections from four tumour-bearing animals show that glioma cells associate with every type of vessel ( j ). In vivo visualization of eGFP-expressing human glioma cells implanted in the cerebrum of immunodeficient mice found invading along the vasculature outlined by tetramethylrhodamine-dextran (TRITC-dex). Arterioles show divergent and venules show convergent blood flow at branch points (arrows in k , o , p ). Perivascular glioma cells can associate with capillaries ( n ), penetrating arterioles ( o ), penetrating venules ( p ). Scale bar, 20 μm. Statistical data: ( a , d ) n =4 animals; ( b ) n =5 animals; ( c ) n =7 animals; ( f ) quantification for n =4 D54 animals, n =3 GBM22 and GBM14 animals; ( g – m ) n =9 animals; ( n – p ) n =34 animals. Full size image Most D54 glioma cells associated with capillaries (<7 μm diameter) that accounted for 47.5% of the total vessel area. About one third of the cells were attached to the penetrating arterioles or collecting veins (7–35 μm diameter, 51% of the total vessel area). Only few cells contacted large arteries or veins (>35 μm diameter) ( Fig. 1g–j ), which represented only 1.6% of the total vessel area measured. Thus, while the low occupancy of large vessels reflects the low occurrence of these vessels, there might be a preference of glioma cells for capillaries over arterioles/venules. Next, we asked whether glioma cells preferentially associate with vessels carrying arterial as opposed to venous blood. Arteries (35–100 μm) and arterioles (7–35 μm) contain contractile VSMCs that regulate vascular tone, and larger arteries have an internal elastic lamina [23] , [24] . Cerebral venules and large veins lack VSMCs and the ability to actively constrict and dilate. All vessels are non-selectively labelled with the endothelial marker CD31 ( Fig. 1a–i ). To identify arterioles/arteries, we used either alpha smooth muscle actin, present in the VSMCs, or Alexa Fluor 633 hydrazide dye, which binds to the elastin found only in arteries/arterioles ≥10 μm in diameter [25] . Representative examples of each vessel type associated with glioma cells are depicted in Fig. 1g–I,k–m and Fig. 2a–c . Quantitative analysis showed 54.46% covering venules/veins over 10 μm and 36.28% associating with arterioles/arteries over 10 μm ( Fig. 1j ). For the 9.25% of vessels between 7 and 10 μm, we were unable to differentiate between arterioles and venules since they lack elastin that is bound by the hydrazide dye ( Fig. 1j ). 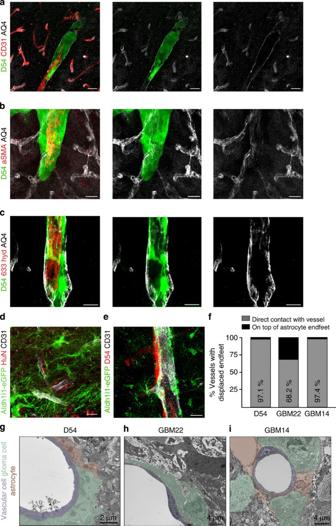Figure 2: Perivascular glioma cells can displace astrocytic endfeet along the vasculature. Immunofluorescence of CD31 (PECAM), aquaporin-4 (AQ4) and eGFP-expressing human glioma cells (D54) implanted in the cerebrum of immunodeficient mice show displacement of the astrocyte endfeet by tumour cells from the vessels in general (a) and from arterioles/arteries labelled with either αSMA (b) or Alexa Fluor 633 hydrazide (633 hyd) (c). This could be confirmed by implanting patient-derived xenograft tumours labelled with human nuclei (HuN) (d) or TdTomato-expressing human glioma cells (D54) (e) into the cerebrum ofAldh1l1-eGFPimmunodeficient mice allowing visualization of astrocyte endfeet independent of AQ4 expression. Perivascular glioma cells can intercalate between endothelial cells and astrocytic endfeet (a,c) or completely displace the astrocytic endfeet from the vascular surface (b). EM (g–i) shows that perivascular astrocytes (brown) are less electron dense than perivascular human glioma cells (green), which can displace astrocytic endfeet, allowing for physical contact with the endothelial cell (g–i) or can sometimes sit on top of the astrocyte endfeet (i). Black font was used to describe white labels in confocal images. See (f) for quantification (n=34 vessels forD54;n=44 forGBM22;n=38 forGBM14). Scale bar, 20 μm (a–e); 2 μm (g), 4 μm (h,i). Statistical data: (a–c)n=18 animals; (d)n=12; (e)n=5 animals; (g)n=3 animals, (h)n=2 animals, (i)n=2 animals. Figure 2: Perivascular glioma cells can displace astrocytic endfeet along the vasculature. Immunofluorescence of CD31 (PECAM), aquaporin-4 (AQ4) and eGFP-expressing human glioma cells ( D54 ) implanted in the cerebrum of immunodeficient mice show displacement of the astrocyte endfeet by tumour cells from the vessels in general ( a ) and from arterioles/arteries labelled with either αSMA ( b ) or Alexa Fluor 633 hydrazide (633 hyd) ( c ). This could be confirmed by implanting patient-derived xenograft tumours labelled with human nuclei (HuN) ( d ) or TdTomato-expressing human glioma cells ( D54 ) ( e ) into the cerebrum of Aldh1l1-eGFP immunodeficient mice allowing visualization of astrocyte endfeet independent of AQ4 expression. Perivascular glioma cells can intercalate between endothelial cells and astrocytic endfeet ( a , c ) or completely displace the astrocytic endfeet from the vascular surface ( b ). EM ( g – i ) shows that perivascular astrocytes (brown) are less electron dense than perivascular human glioma cells (green), which can displace astrocytic endfeet, allowing for physical contact with the endothelial cell ( g – i ) or can sometimes sit on top of the astrocyte endfeet ( i ). Black font was used to describe white labels in confocal images. See ( f ) for quantification ( n =34 vessels for D54 ; n =44 for GBM22 ; n =38 for GBM14 ). Scale bar, 20 μm ( a – e ); 2 μm ( g ), 4 μm ( h , i ). Statistical data: ( a – c ) n =18 animals; ( d ) n =12; ( e ) n =5 animals; ( g ) n =3 animals, ( h ) n =2 animals, ( i ) n =2 animals. Full size image To complement these studies, we also assessed vessel preference of invading glioma cells in vivo by two-photon imaging. A craniotomy was performed in tumour-implanted mice and the vasculature was highlighted by tail vein injection of tetramethylrhodamine (TRITC)-dextran. The direction of the blood flow and size of the vessel were used to identify the vessel type; arterioles show divergent and venules show convergent blood flow at branch points ( Fig. 1n–p ). Taken together, these studies suggest that a vast majority of gliomas associate with blood vessel along the entire vascular tree with a clear preference for small calibre capillaries. Glioma cells displace astrocyte endfeet from the vasculature The brain’s vascular surface is over 99% covered by astrocytic endfeet [2] , which are anchored to the basement membrane of the endothelial cells via integrin, dystroglycan and agrin [6] leaving only a minute Virchow–Robin space filled with interstitial fluid that is part of the ‘glymphatic’ system [26] . Hence, as glioma cells invade along blood vessels, astrocytic endfeet may pose an obstacle to cell movement. To examine the physical relationship between endfeet, gliomas and blood vessels, we used cell type-specific markers on histological sections. As illustrated in Fig. 2 , the normal interaction between the astrocytic endfeet and vasculature is frequently disrupted by the presence of perivascular glioma cells either by the physical displacement of the astrocytic endfeet labelled with aquaporin-4 ( Fig. 2a,c ) or by the elimination of the endfeet altogether ( Fig. 2b ), presumably through process retraction as previously reported [19] . To ensure that the latter was not due to a loss of aquaporin-4 protein in the membrane, we repeated these studies using an immunodeficient reporter mouse with expression of eGFP under the astrocyte-specific Aldh1l1 promoter and tumour cells either expressing the red fluorescent TdTomato (D54) or detected by antibody staining against human nuclei (GBM). Immunohistochemistry from these animals again show that glioma cells indeed displaced the astrocytic endfeet away from the vasculature and are in direct contact with endothelial cells ( Fig. 2d,e , Supplementary Fig. 2 ). As expected, vessels not occupied by glioma cells remain covered by astrocytic endfeet ( Supplementary Fig. 2c ). To study the displacement of astrocytic endfeet by individual glioma cells at even higher resolution, we employed electron microscopy (EM) ( Fig. 2g–i , Supplementary Figs 3–5 ). Criteria for the distinction of glioma cells and astrocyte processes included the different electron densities of glioma cells and astrocytes ( Supplementary Fig. 4e ). A higher electron density and hence darker appearance of the glioma cytoplasm is due to a rougher endoplasmic reticulum [27] . Glioma cells also showed a high nucleus to cytoplasm ratio with large, often convoluted or segmented nuclei and multiple nucleoli. Euchromatin is more abundant than heterochromatin resulting in an even higher electron density of the glioma nucleus [28] . In contrast, astrocyte endfeet are characterized by a less electron-dense (lighter) cytoplasm with internal substructures of filamentous networks and bundles of glial filaments [29] ( Supplementary Fig. 4e ). We found glioma cells, distinguished from astrocytes by increased electron density and enlarged nuclei ( Fig. 2g–i , Supplementary Figs 3–5 , confirmed by a clinical pathologist), displacing the astrocyte endfeet from the endothelial wall in a majority of the analysed vessels of D54 -, GBM22 - and GBM14 -implanted mice ( Fig. 2f–i , see Supplementary Figs 3–5 for additional examples and quantification). However, on some vessels, glioma cells were in close proximity of the vessel wall, but still separated by the astrocytic endfeet ( Fig. 2f,i , Supplementary Fig. 5f ). Taken together, these studies illustrate that glioma cells can gain direct access to the abluminal side of cerebral vessels through the displacement of astrocytic endfeet. Vessel co-option by glioma cells breaches the BBB Development of the BBB precedes astrocyte development and is induced by pericytes [30] , [31] , yet maintenance of an intact barrier relies on soluble factors released by astrocytes and persistent contact between astrocytes and endothelial cells [5] , [32] . Accordingly, pathological conditions that compromise astrocytes are also present with an impaired BBB [4] . A leaky BBB is also typical for newly generated glioma vasculature that lacks TJs [33] . This can be readily demonstrated by permeation of Evan’s blue from the bloodstream into the brain parenchyma surrounding a large tumour mass ( Fig. 3a ). 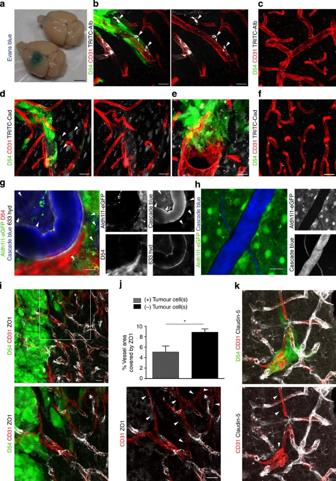Figure 3: Perivascular glioma cell co-option causes a breakdown of the BBB. The tracer, Evans blue, permeates into the brain parenchyma in tumour-bearing (n=3 animals) (bottom), but not in sham mice 3 weeks post surgery (n=3 animals) (top), Scale bar, 5 mm. (a) Immunofluorescence of CD31 and intravenously injected tracers, tetramethylrhodamine-albumin (TRITC-alb, white) or -cadaverine (TRITC-cad, white), and implanted eGFP-expressing human glioma cells (D54) allow analysis of tracer leakage in relation to tumour burden. The large MW 70 kDa TRITC-albumin (b), as well as the small MW 950 kDa TRITC-cadaverine (d) can be found outside the vasculature (arrows) (b–f,Supplementary Fig. 6). Note that leaked TRITC-cadaverine is taken up by nearby neurons (arrows) (d,e). No extravasation was seen in the absence of tumour cells (c,f). To assess extravasation of the tracer Cascade Blue (MW 10 kDa),Aldh1l1-eGFP-scid(eGFP) immunodeficient mice, which were previously implanted with TdTomato-expressing human glioma cells (D54), were retroorbitally injected with Alexa Fluor 633 hydrazide dye (633 hyd) and Cascade Blue (g,h). Accumulation of Cascade Blue occurs in the brain’s parenchyma indicating breakdown of the BBB, where perivascular astrocytes have been displaced by glioma cell co-option (g). Vessels lacking tumour cells do not show extravasation of the dye (h). Immunohistochemistry for the TJ proteins ZO-1 (i) and claudin-5 (k) show that these protein are lost from endothelial cells labelled with CD31 where tumour cells are present (enlarged panel, arrows), but colocalize with endothelial cells in tissue that has not been co-opted. Quantification of ZO-1 shows reduction of vessel coverage in areas co-opted by glioma cells. 8.86±0.64% vessel area is covered by ZO-1 in control images, whereas this number was reduced to 5.1±1.11% in areas where vessels were co-opted by tumour cells (n=9 images each for control and tumour-covered vessels from three animals, pairedt-test directly comparing control and tumour images in the same slice,P=0.037, *represents statistical significance with a p-value <0.05, error bars refer to s.e.m.) (j). Black font was used to describe white labels in confocal images. Scale bar, 20 μm. Statistical data: (b,c)n=10 animals; (d–f)n=7 animals; (g)n=2 animals; (h)n=4 animals; (i,k)n=6 animals. Figure 3: Perivascular glioma cell co-option causes a breakdown of the BBB. The tracer, Evans blue, permeates into the brain parenchyma in tumour-bearing ( n =3 animals) (bottom), but not in sham mice 3 weeks post surgery ( n =3 animals) (top), Scale bar, 5 mm. ( a ) Immunofluorescence of CD31 and intravenously injected tracers, tetramethylrhodamine-albumin (TRITC-alb, white) or -cadaverine (TRITC-cad, white), and implanted eGFP-expressing human glioma cells ( D54 ) allow analysis of tracer leakage in relation to tumour burden. The large MW 70 kDa TRITC-albumin ( b ), as well as the small MW 950 kDa TRITC-cadaverine ( d ) can be found outside the vasculature (arrows) ( b – f , Supplementary Fig. 6 ). Note that leaked TRITC-cadaverine is taken up by nearby neurons (arrows) ( d , e ). No extravasation was seen in the absence of tumour cells ( c , f ). To assess extravasation of the tracer Cascade Blue (MW 10 kDa), Aldh1l1-eGFP-scid (eGFP) immunodeficient mice, which were previously implanted with TdTomato-expressing human glioma cells ( D54 ), were retroorbitally injected with Alexa Fluor 633 hydrazide dye (633 hyd) and Cascade Blue ( g , h ). Accumulation of Cascade Blue occurs in the brain’s parenchyma indicating breakdown of the BBB, where perivascular astrocytes have been displaced by glioma cell co-option ( g ). Vessels lacking tumour cells do not show extravasation of the dye ( h ). Immunohistochemistry for the TJ proteins ZO-1 ( i ) and claudin-5 ( k ) show that these protein are lost from endothelial cells labelled with CD31 where tumour cells are present (enlarged panel, arrows), but colocalize with endothelial cells in tissue that has not been co-opted. Quantification of ZO-1 shows reduction of vessel coverage in areas co-opted by glioma cells. 8.86±0.64% vessel area is covered by ZO-1 in control images, whereas this number was reduced to 5.1±1.11% in areas where vessels were co-opted by tumour cells ( n =9 images each for control and tumour-covered vessels from three animals, paired t -test directly comparing control and tumour images in the same slice, P =0.037, *represents statistical significance with a p-value <0.05, error bars refer to s.e.m.) ( j ). Black font was used to describe white labels in confocal images. Scale bar, 20 μm. Statistical data: ( b , c ) n =10 animals; ( d – f ) n =7 animals; ( g ) n =2 animals; ( h ) n =4 animals; ( i , k ) n =6 animals. Full size image In light of the demonstrated displacement of astrocytes by perivascular glioma cells, we asked if focal disruption of the normal astrocyte–endothelial cell interactions along the existing vessels was sufficient to breach the BBB. Therefore, we examined the leakage of TRITC-albumin (MW 70 kDa) from blood vessels distant from the D54 -tumour mass and associated with only few glioma cells. As expected, the main tumour mass, where angiogenesis leads to the formation of naïve and leaky immature microvessels, showed extensive extravasation of the TRITC-albumin from the vasculature ( Supplementary Fig. 6 ). However, even at distant sites where vessels were associated with only small groups of cells or even just a single glioma cell, the dye was still found outside the lumen of the vasculature suggesting a focal breach of the BBB ( Fig. 3b ). Surprisingly, just a few cells were sufficient to cause albumin leakage. No leakage was observed in the cortical areas lacking tumour in the same animal ( Fig. 3c ). We obtained similar results with a second, much smaller, permeability marker, TRITC-cadaverine (MW 950 Da) that is taken up by surrounding neurons [30] ( Fig. 3d,e ). Again, no leakage was observed in glioma-free vessels in the same animals ( Fig. 3f ). Animals intracranially implanted with non-malignant primary mouse glial cells obtained from Aldh1l1-eGFP -scid mice were retroorbitally injected with cadaverine-Alexa555, Evans blue and albumin-Alexa555 3, 7 and 14 days later. Dye leakage was restricted to the area surrounding the needle tract at all time points and decreased over time suggesting that the injury inflicted by the needle healed and non-malignant glial cells do not cause breach of the BBB ( Supplementary Fig. 7 ). We also examined BBB integrity in vivo , using a 10 kDa permeability marker, Cascade Blue, injected retroorbitally. Two-photon imaging revealed clouds of Cascade Blue emanating from vessels where invading gliomas had displaced the astrocytic endfeet ( Fig. 3g , Supplementary Fig. 6c ), yet no leakage was observed along glioma-free vessels ( Fig. 3h ). Endothelial TJs form the physical barrier limiting diffusion of blood-borne molecules into the brain’s parenchyma and are characterized by the presence of proteins such as zonula occludens-1 (ZO-1) and claudin-5. The presence of single tumour cells can reduce the expression of ZO-1 ( Fig. 3i,j ). Similarly, claudin-5 is abundant along vessels lacking tumour cells, but is largely diminished where tumour cells contact the vasculature ( Fig. 3k ). Taken together, these data suggest that the focal displacement of an astrocyte endfeet by a single or few glioma cells is sufficient to open the BBB presumably through a loss of TJs. Glioma cells cause loss of astrocyte–vascular coupling Release of vasoactive molecules by astrocytic endfeet onto blood vessels, also called gliovascular coupling, causes local changes in the cerebral blood flow in response to neuronal activity [7] . Specifically, activation of astrocytic G-protein-coupled receptors (GPCRs) causes an increase in [Ca 2+ ] i , and activation of phospholipase A 2 , which converts membrane phospholipids into AA. AA can be either released from the astrocyte to be converted into 20-HETE in the VSMC causing vasoconstriction or metabolized into PGE 2 , which dilates vessels. Ca 2+ is the cellular signal that precedes a vessel diameter change and the type of response, dilation or constriction, can be modulated by the brain’s metabolism [34] (schematically depicted in Fig. 8). Central to the astrocyte-mediated control of blood flow is the presence of endfeet on the vasculature. Since we found astrocytic endfeet along arterioles frequently displaced from the VSMCs by perivascular glioma cells ( Figs 2b,c and 3g , Supplementary Figs 2–5 ), we questioned whether vascular coupling was altered. To answer this, we first used a pharmacological approach to selectively stimulate astrocytes and assessed responses of the arterioles. We bath applied two drugs known to selectively increase [Ca 2+ ] i in astrocytes, namely trans -ACPD (t-ACPD) and norepinephrine (NE) [11] , [34] , [35] to acute brain slices and measured the vessel diameter change by video microscopy for arterioles identified by a thickened vessel wall indicating the presence of a VSMC layer with D54 ((+)tumour cell(s)) or without perivascular glioma cells ((−) tumour cell(s)). For all experiments, diameter changes in response to t-ACPD and NE were assessed at high (95%) and low (20%) oxygen concentrations, as these oxygen concentrations have been shown to cause opposite vascular responses due to the limitation of 20-HETE and nitric oxide production by limited oxygen amounts [7] , [34] . In agreement with previous studies [11] , [34] , application of t-ACPD caused vasodilatation (O 2 low , n= 12) or vasoconstriction (O 2 high , n =20) in tumour-free vessels ( Fig. 4a–c ). Similarly, NE application induced constriction (O 2 high , n =18) or dilation (O 2 low , n =22) in glioma-free arterioles ( Fig. 4d–f ). In contrast, arterioles encased by glioma cells showed a significant decrease in vessel response after t-ACPD (O 2 low : n =9, two-tailed unpaired t -test, P =0.012; O 2 high : n =16, two-tailed Mann–Whitney test, P =0.0032) ( Fig. 4a–c ) or NE application (O 2 high : n =18, two-tailed unpaired t -test, P =0.0049; O 2 low : n =21, two-tailed unpaired t -test, P =0.01) ( Fig. 4d–f ). 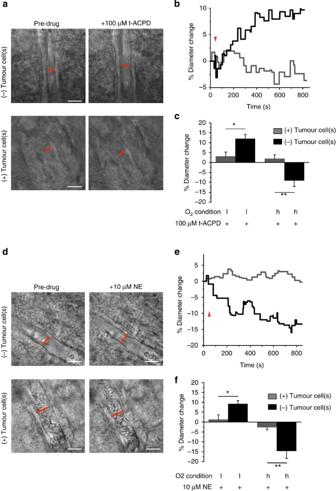Figure 4: Loss of astrocyte–vascular coupling following vessel co-option by gliomas. (a) DIC images of vessels without (top) or with (bottom) perivascular glioma cells before and after application of 100 μM t-ACPD. Perivascular glioma cell presence was verified by eGFP fluorescence. (b) Changes in vessel diameter for an arteriole associated (grey) and not associated (black) with perivascular glioma cells over the course of one experiment when exposed to 100 μM t-ACPD (arrowhead). (c) Average change in the vessel diameters observed at high (h) (95%) and low (l) (20%) oxygen for vessels associated (grey) and not associated (black) with glioma cells when exposed to 100 μM t-ACPD. (d) DIC images of vessels without (top) or with (bottom) perivascular glioma cells before and after application of 10 μM NE. Perivascular glioma cell presence was verified by eGFP fluorescence. (e) Changes in vessel diameter for an arteriole associated (grey) and not associated (black) with perivascular glioma cells over the course of one experiment when exposed to 10 μM NE (arrowhead). (f) Average change in the vessel diameters observed at high (h) (95%) and low (l) (20%) oxygen for vessels associated (grey) and not associated (black) with glioma cells when exposed to 10 μM NE. For experiments performed at low oxygen concentrations, arterioles were preconstricted with 125 nM U46619 for 20 min. Statistical data provided in results section, error bars refer to s.e.m. *P-value <0.05, **P-value <0.01. Scale bar, 20 μm. Figure 4: Loss of astrocyte–vascular coupling following vessel co-option by gliomas. ( a ) DIC images of vessels without (top) or with (bottom) perivascular glioma cells before and after application of 100 μM t-ACPD. Perivascular glioma cell presence was verified by eGFP fluorescence. ( b ) Changes in vessel diameter for an arteriole associated (grey) and not associated (black) with perivascular glioma cells over the course of one experiment when exposed to 100 μM t-ACPD (arrowhead). ( c ) Average change in the vessel diameters observed at high (h) (95%) and low (l) (20%) oxygen for vessels associated (grey) and not associated (black) with glioma cells when exposed to 100 μM t-ACPD. ( d ) DIC images of vessels without (top) or with (bottom) perivascular glioma cells before and after application of 10 μM NE. Perivascular glioma cell presence was verified by eGFP fluorescence. ( e ) Changes in vessel diameter for an arteriole associated (grey) and not associated (black) with perivascular glioma cells over the course of one experiment when exposed to 10 μM NE (arrowhead). ( f ) Average change in the vessel diameters observed at high (h) (95%) and low (l) (20%) oxygen for vessels associated (grey) and not associated (black) with glioma cells when exposed to 10 μM NE. For experiments performed at low oxygen concentrations, arterioles were preconstricted with 125 nM U46619 for 20 min. Statistical data provided in results section, error bars refer to s.e.m. * P -value <0.05, ** P -value <0.01. Scale bar, 20 μm. Full size image Slices obtained from D54-GCaMP3-GFP tumours bearing a genetically encoded Ca 2+ sensor showed no significant Ca 2+ increase induced by t-ACPD or NE in glioma cells ( Supplementary Fig. 8a ) assuring that the effects of both drugs are targeted to astrocytes as previously demonstrated [11] , [34] , [35] . To further ensure that the observed lack in vessel response is indeed due to diminished astrocyte–vascular coupling and not caused by unspecific effects of the drugs on other cell types, we stimulated single astrocytes surrounding vessels with or without glioma cells by uncaging [Ca 2+ ] i after loading acute brain slices of tumour-bearing animals with DMNPE-4 caged Ca 2+ (ref. 36 ). In control slices derived either from naïve animals or from brain regions devoid of tumour, uncaging Ca 2+ corresponds to an increase in Ca 2+ detected by the Ca 2+ -indicator dye Fluo-4, which was followed by either constriction or dilation of the nearby arteriole ( Fig. 5a–c,g,h ; Supplementary Movies 1,2 ). 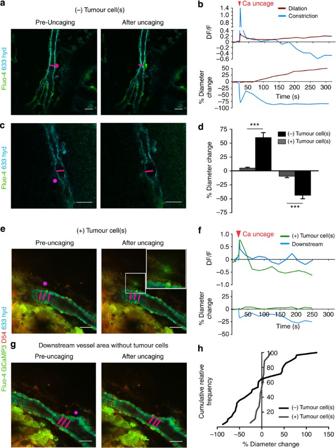Figure 5: Vascular responses to Ca2+uncaging in astrocytes is impaired in vessels co-opted by glioma cells. [Ca2+]iuncaging in an astrocyte endfeet or cell body close to an arteriole free of glioma cells leads to either constriction (a) or dilation (c) of the vessel. The vessel response is preceded by a rise in [Ca2+]i(b,d). The pink spot indicates the location of Ca2+ uncaging. Measurement of the Ca2+response was performed in this region or in an immediate adjacent region. Vessels encased by glioma cells do not respond to Ca2+uncaging in nearby astrocytes (e,f). Stimulation of astrocytes in tumour-free areas of the same vessel (downstream vessel area) causes constriction showing that the lack of response is specific for areas covered by glioma cells (f,g). The cumulative relative frequency distribution shows a wide range of dilatory or constricting vessel responses in controls, whereas most vessels associated with glioma do not respond or do so to a lesser extent (h). Statistical data in (d): control dilating vessels, 60.05±8.899%,n=10 vessels, tumour dilating, 5.18±1.493,n=8, two-tailed unpairedt-test,P≤0.0001; control constricting vessels, −43.51±6.283%n=18 vessels, glioma constricting, −9.389±2.611%,n=9. Two-tailed unpairedt-test,P≤0.001, error bars refer to s.e.m., *P-value <0.05, **P-value <0.01, ***P-value <0.001. Scale bar, 20 μm. Figure 5: Vascular responses to Ca 2+ uncaging in astrocytes is impaired in vessels co-opted by glioma cells. [Ca 2+ ] i uncaging in an astrocyte endfeet or cell body close to an arteriole free of glioma cells leads to either constriction ( a ) or dilation ( c ) of the vessel. The vessel response is preceded by a rise in [Ca 2+ ] i ( b , d ). The pink spot indicates the location of Ca2+ uncaging. Measurement of the Ca 2+ response was performed in this region or in an immediate adjacent region. Vessels encased by glioma cells do not respond to Ca 2+ uncaging in nearby astrocytes ( e , f ). Stimulation of astrocytes in tumour-free areas of the same vessel (downstream vessel area) causes constriction showing that the lack of response is specific for areas covered by glioma cells ( f , g ). The cumulative relative frequency distribution shows a wide range of dilatory or constricting vessel responses in controls, whereas most vessels associated with glioma do not respond or do so to a lesser extent ( h ). Statistical data in ( d ): control dilating vessels, 60.05±8.899%, n =10 vessels, tumour dilating, 5.18±1.493, n =8, two-tailed unpaired t -test, P ≤0.0001; control constricting vessels, −43.51±6.283% n =18 vessels, glioma constricting, −9.389±2.611%, n =9. Two-tailed unpaired t -test, P ≤0.001, error bars refer to s.e.m., * P -value <0.05, ** P -value <0.01, *** P -value <0.001. Scale bar, 20 μm. Full size image This response occurred within seconds on a faster time scale than the response after drug application, which is likely due to the slow perfusion and diffusion of the drugs into the slice. In contrast, Ca 2+ uncaging in astrocytes close to the vessels co-opted by D54 glioma cells failed to respond ( Fig. 5d–f,h ) indicating that astrocyte-derived signals do not reach the vasculature. However, the same vessels responded if astrocytes were stimulated in areas that were not covered by glioma cells ( Fig. 5f,g ). Taken together, these data show that the presence of perivascular glioma cells is sufficient to disrupt astrocyte-mediated gliovascular coupling (schematically depicted in Fig. 8). Perivascular glioma cells do not compromise VSMC function Although the above data suggest that the displacement of the astrocytic endfeet from the vessel is responsible for a loss of vasoregulation by astrocytes, it is also possible that the presence of glioma cells may have impaired the function of the arterial smooth muscle cells. To address this possibility, we compared vessel responses of arterioles associated and those not associated with glioma cells after bath application of drugs known to directly target VSMCs. We applied (a) the thromboxane A 2 agonist U46619, a stable synthetic analogue of PGH 2 , which constricts parenchymal arteries by binding to TXA 2 receptors on VSMCs [8] , [37] , [38] , (b) K + , which produces significant vasoconstriction by activating VSMC voltage-dependent Ca 2+ channels [9] and (c) endothelin-1 (ET-1), a potent vasoconstrictor [39] released by vascular endothelial cells that binds to the endothelin receptor found on VSMCs. These three vasoconstrictive agents showed no significant difference whether applied to glioma-associated or glioma-free vessels ( Fig. 6a,b ). 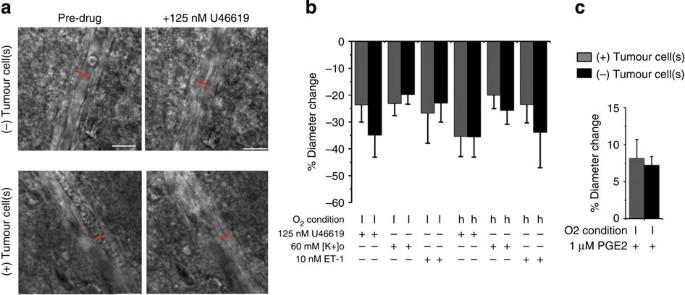Figure 6: Perivascular glioma cells do not compromise vascular smooth muscle cell function. DIC images of vessels without (top) or with (bottom) perivascular glioma cells before and after application of 125 nM U46619. Perivascular glioma cell presence was verified by eGFP fluorescence (a). Average change in vessel diameters observed at high (h) (95%) and low (l) (20%) oxygen for vessels associated (grey) and not associated (black) with glioma cells when exposed to 125 nM U46619, 60 mM [K+]o, 10 nM ET-1 (b) and 1 μM PGE2(c). For 1 μM PGE2, arterioles were preconstricted with 125 nM U46619 for 20 min. Statistical data as follows: 20% oxygen. 125 nM U46619: (+) tumour cell(s)n=11, (−) tumour cell(s)n=11, two-tailed Mann–Whitney test,P=0.40; 60 mM [K+]o: (+) tumour cell(s)n=10, (−) tumour cell(s)n=9, two-tailed unpairedt-test,P=0.57; 10 nM ET-1: (+) tumor cell(s)n=8, (−) tumour cell(s)n=9, two-tailed unpairedt-test,P=0.78; 1 μM PGE2: (+) tumour cell(s)n=14, (−) tumour cell(s)n=21, two-tailed unpairedt-test,P=0.72. 95% oxygen. 125 nM U46619: (+) tumour cell(s)n=14. (−) tumour cell(s)n=12, two-tailed unpairedt-test,P=0.99; 60 mM [K+]o: (+) tumour cell(s)n=11, (−) tumour cell(s)n=19, two-tailed Mann–Whitney Test,P>0.9999; 10 nM ET-1: (+) tumour cell(s)n=7, (−) tumour cell(s)n=9, two-tailed unpairedt-test,P=0.48). Error bars refer to s.e.m. Scale bar, 20 μm. Figure 6: Perivascular glioma cells do not compromise vascular smooth muscle cell function. DIC images of vessels without (top) or with (bottom) perivascular glioma cells before and after application of 125 nM U46619. Perivascular glioma cell presence was verified by eGFP fluorescence ( a ). Average change in vessel diameters observed at high (h) (95%) and low (l) (20%) oxygen for vessels associated (grey) and not associated (black) with glioma cells when exposed to 125 nM U46619, 60 mM [K + ] o , 10 nM ET-1 ( b ) and 1 μM PGE 2 ( c ). For 1 μM PGE 2 , arterioles were preconstricted with 125 nM U46619 for 20 min. Statistical data as follows: 20% oxygen. 125 nM U46619: (+) tumour cell(s) n =11, (−) tumour cell(s) n =11, two-tailed Mann–Whitney test, P =0.40; 60 mM [K + ] o : (+) tumour cell(s) n =10, (−) tumour cell(s) n =9, two-tailed unpaired t -test, P =0.57; 10 nM ET-1: (+) tumor cell(s) n =8, (−) tumour cell(s) n =9, two-tailed unpaired t -test, P =0.78; 1 μM PGE 2 : (+) tumour cell(s) n =14, (−) tumour cell(s) n =21, two-tailed unpaired t -test, P =0.72. 95% oxygen. 125 nM U46619: (+) tumour cell(s) n =14. (−) tumour cell(s) n =12, two-tailed unpaired t -test, P =0.99; 60 mM [K + ] o : (+) tumour cell(s) n =11, (−) tumour cell(s) n =19, two-tailed Mann–Whitney Test, P >0.9999; 10 nM ET-1: (+) tumour cell(s) n =7, (−) tumour cell(s) n =9, two-tailed unpaired t -test, P =0.48). Error bars refer to s.e.m. Scale bar, 20 μm. Full size image Similarly, the vasodilator PGE 2 , which binds receptors of the prostaglandin receptor family on VSMCs [40] , dilated arterioles that were preconstricted with U46619 as previously described [34] with no significant difference whether gliomas were present or not ( Fig. 6c ). The lack of a difference in the responsiveness of these two populations of vessels suggests that the perivascular glioma cells do not affect the function of the VSMC. Perivascular glioma cells assume control of vasculature tone Once gliomas have displaced astrocytes from the vessel, they often completely encase the blood vessel ( Figs 1a and 2b,c ). This begs the question whether glioma cells are now also in a position to actively control vessel tone using the same or different mechanisms employed normally by astrocytes. Previous studies report a significant dilation of vessels within the main tumour mass [21] , which we could confirm in our animal models ( Supplementary Fig. 9a,b ). However, preexisting vessels with glioma cells do not have significantly larger vessel diameters overall ( Supplementary Fig. 9c ). Nonetheless, glioma cells might regulate vascular tone upon stimulation. To examine a potential glioma-mediated vascular regulation, we exploited both Ca 2+ photo-uncaging from glioma cells and the use of the protease-activated receptor 1 (PAR1). PAR1 is a GPCR that is highly expressed in glioma cells where its activation causes an increase in [Ca 2+ ] i [41] . Natural ligands for PAR1 include thrombin and plasmin [42] , both found within the vasculature. Bath application of the selective PAR1 agonist, TFLLR, to control or glioma-bearing brain slices did not cause a detectable increase in [Ca 2+ ] i in astrocytes ( Supplementary Fig. 8c ). Accordingly, arterioles lacking perivascular glioma cells ( n =10) caused no change in vessel diameter ( Fig. 7a–c , Supplementary Fig. 8b , Supplementary Movie 3 ). In contrast, in arterioles completely surrounded by perivascular glioma cells, TFLLR caused a significant vasoconstriction (( n =9), two-tailed unpaired t -test, P =<0.0001) ( Fig. 7a–c , Supplementary Movie 4 ). The use of GCamp3-expressing glioma cells allowed us to examine the temporal relationship of the PAR1-mediated Ca 2+ increases and the ensuing vessel constriction because an increase in GFP fluorescence corresponds to increases in [Ca 2+ ] i . A pronounced Ca 2+ increase preceded vasoconstriction of the arteriole ( Fig. 7b,c , Supplementary Movie 4 ), similar to previous reports in astrocytes [35] . Accordingly, we could induce a vascular response by uncaging [Ca 2+ ] i in glioma cells that are in contact with arterioles ( Fig. 7d,e , Supplementary Fig. 8c , Supplementary Movie 5 ). In cortical astrocytes, K + release via Ca 2+ -activated BK channels has been shown to control cerebral blood vessels, dictating whether vasoconstriction or vasodilation occurs depending on the resulting extracellular concentration of K + (refs 8 , 9 ). Glioma cells abundantly express two Ca 2+ -activated K + channels, BK and IK [43] , [44] , which each may mediate K + efflux following PAR1-induced [Ca 2+ ] i rises. To examine this possibility, we repeated the above PAR1-activation experiments in the combined presence of the selective inhibitors paxilline and Tram-34 that specifically block BK and IK channels, respectively. Again, arterioles lacking perivascular glioma cells did not alter their vessel diameter following PAR1 activation ( n =17) ( Fig. 7a ). However, arterioles with perivascular glioma cells constricted significantly less ( n =15) ( Fig. 7a ) in the presence of these K + channel blockers suggesting that efflux of K + , from the glioma cells, contributed to glioma-mediated vasoregulation (one-tailed unpaired t -test with Welch correction, P =0.044, schematically depicted in Fig. 8). In cortical astrocytes, the concentration of K + released determines whether vessels dilate or constrict [35] . Therefore, it is conceivable that glioma cells similarly are capable of causing either constrictions or dilation. 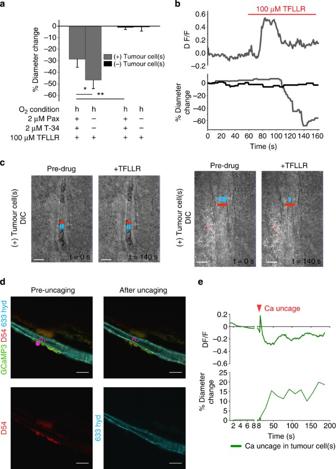Figure 7: Perivascular glioma cells can hijack control over vasculature tone similar to astrocytes. Average change in vessel diameters observed in high (h) (95%) oxygen for vessels associated (grey) and not associated (black) with glioma cells when exposed to 100 μM TFLLR or 100 μM TFLLR+2 μM paxilline (Pax)+2 μM Tram-34 (a). Changes in the vessel diameter for an arteriole associated (grey) and not associated (black) with perivascular glioma cells over the course of one experiment when exposed to 100 μM TFLLR. Changes in Ca2+(ΔF/F) in perivascular GCamp3-GFP-expressing glioma cells were simultaneously measured over the course of this experiment (b). DIC images of vessel associated with glioma cells ((−) tumour cells) before and after sufficient exposure to 100 μM TFLLR (left), ((+)tumour cells) before and at most constricted time point after application of 100 μM TFLLR (right), red lines indicate position of diameter measurement and vessel diameter before drug application, blue arrows indicate vessel diameter, scale bar, 10 μm (c). Statistical data provided in results section, error bars refer to s.e.m., *P-value <0.05, **P-value <0.01. Acute slices from mice bearing GCamp3-GFP-expressing D54 gliomas that also expressed the red fluorescent protein tdTomato were loaded with DMNPE-4 caged Ca2+. [Ca2+]iuncaging in TdTomato-positive glioma cells located at arterioles resulted in vascular responses (n=3), this example shows a dilation (d) scale bar, 20 μm. Traces showing a fast [Ca2+]Iincrease preceding the vascular response and slower oscillations at later time points. Data were corrected for dye bleaching using the bleach correction macro for ImageJ (e). Figure 7: Perivascular glioma cells can hijack control over vasculature tone similar to astrocytes. Average change in vessel diameters observed in high (h) (95%) oxygen for vessels associated (grey) and not associated (black) with glioma cells when exposed to 100 μM TFLLR or 100 μM TFLLR+2 μM paxilline (Pax)+2 μM Tram-34 ( a ). Changes in the vessel diameter for an arteriole associated (grey) and not associated (black) with perivascular glioma cells over the course of one experiment when exposed to 100 μM TFLLR. Changes in Ca 2+ (Δ F/F ) in perivascular GCamp3-GFP-expressing glioma cells were simultaneously measured over the course of this experiment ( b ). DIC images of vessel associated with glioma cells ((−) tumour cells) before and after sufficient exposure to 100 μM TFLLR (left), ((+)tumour cells) before and at most constricted time point after application of 100 μM TFLLR (right), red lines indicate position of diameter measurement and vessel diameter before drug application, blue arrows indicate vessel diameter, scale bar, 10 μm ( c ). Statistical data provided in results section, error bars refer to s.e.m., * P -value <0.05, ** P -value <0.01. Acute slices from mice bearing GCamp3-GFP-expressing D54 gliomas that also expressed the red fluorescent protein tdTomato were loaded with DMNPE-4 caged Ca 2+ . [Ca 2+ ] i uncaging in TdTomato-positive glioma cells located at arterioles resulted in vascular responses ( n =3), this example shows a dilation ( d ) scale bar, 20 μm. Traces showing a fast [Ca 2+ ] I increase preceding the vascular response and slower oscillations at later time points. Data were corrected for dye bleaching using the bleach correction macro for ImageJ ( e ). Full size image Using a clinically relevant mouse model of glioma, which replicates the salient features of the disease including diffuse perivascular invasion [45] , peritumoral excitotoxicity [46] , [47] and seizures [46] , we investigated the interaction of invading glioma cells with host cerebral blood vessels during early stages of disease questioning whether invading perivascular glioma cells may disrupt the astrocyte–vascular contact and in turn compromise their functional interactions. Using brain slices and in vivo imaging, we show that the vast majority of glioma associate with existing vessels and can displace the astrocytic endfeet from the vascular surface. This can cause a loss of endothelial cell TJs resulting in the extravasation of blood-borne molecules such as albumin, cadaverine or cascade blue tracers into the brain’s parenchyma. Vessels occupied by gliomas no longer respond to astrocyte-released vasoregulators. Once vessels are fully encased, gliomas assume the regulation of vascular tone in part through the release of K + via Ca 2+ -activated K + channels. Gliomas are known as highly vascular cancers and past studies have extensively studied glioma-mediated neovascularization and angiogenesis [17] . Glioma-released VEGF incites microvascular proliferation and produce naïve, leaky and dilated blood vessels [48] . Tumour tissue from glioblastoma patients show downregulation of key TJ proteins including claudin−1, −3 and −5 (refs 6 , 49 ), which explains why tumours present with leaky BBBs as also observed in our mouse model. In contrast to previous studies, we examined glioma–vascular interactions at a much earlier disease stage during a period termed vascular co-option, which precedes angiogenesis. Here, invading glioma cells, known to prefer the perivascular space for invasion [20] , wrap themselves around the abluminal surface in a parasitic manner [16] , [18] often fully encasing blood vessels. Our data show that single invading cells or small groups of cells are sufficient to cause a local breach of the BBB. This could be attributed to the physical separation of the endfeet from the vessel surface. Such interdependence had been postulated [50] ; however, a model examining selective astrocytic endfeet separation from the vasculature had not existed. Alternatively, contact and interaction of glioma cells with the vasculature could impair BBB functionality and expression of TJ proteins directly. A lack of pericytes is associated with BBB damage during development and in the aging brain [51] . Furthermore, activation of a proinflammatory cascade in pericytes in response to ApoE4 expression leads to BBB breakdown [52] . For future studies, it will be interesting to examine whether pericytes contribute to BBB breakdown in response to glioma invasion. Irrespective of the cause, this finding is unexpected and exciting, because it suggests that small groups of invading tumour cells are not protected from the reach of chemotherapeutic drugs by the BBB as previously assumed, and aggressive chemotherapy could be considered at early stages of the disease when invasion is still rampant. A second major finding of our study relates to the loss of functional coupling of astrocytes to regional blood flow. We find that the physical displacement of the astrocytic endfeet by gliomas prevents vasoactive molecules from reaching the vascular endothelial cell, while the VSMCs are largely unaffected by the presence of gliomas and still respond to vasoactive molecules directly applied (summarized in Fig. 8 ). We stimulated astrocytic G-protein-coupled receptors using two drugs, t-ACPD and NE, which have previously been shown to selectively induce [Ca 2+ ] i rises in astrocytes [11] , [34] , [35] causing dilation in 20% oxygen and constriction in 95% oxygen. We complemented the pharmacological experiments by directly uncaging [Ca 2+ ] i in single astrocytes close to vessels. Indeed, vessels not occupied by gliomas showed identical responses to those studies previously published refs 11 , 34 , 35 , with either the pharmacological approach or photo-uncaging of Ca 2+ . Remarkably, we found a wide range of constrictions and dilations after Ca 2+ uncaging. This is likely due to different levels of Ca 2+ increases in the astrocytic endfeet as modest increases in Ca 2+ induce dilation whereas larger increases cause constrictions [9] . In addition, the vascular response is dependent on [K + ] o levels. Raising extracellular [K + ] o switches dilation to constriction in brain slices. Indeed, we observed only constrictions when we applied high [K + ] o to slices independent of the oxygen tension. 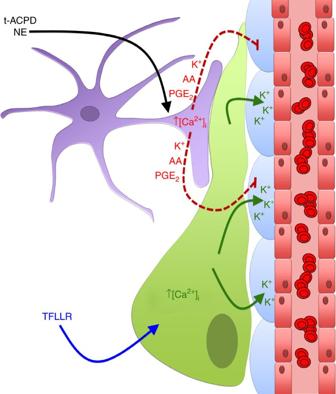Figure 8: Perivascular glioma cells disrupt astrocyte-mediated vascular coupling. The perivascular glioma cell (green) inserts itself between the VSMCs (blue) surrounding the vascular endothelial cells (red), displacing the astrocytic endfeet (purple). Bath application of NE and t-ACPD activates astrocytic G-protein-coupled receptors causing an increase in astrocytic [Ca2+]i. Due to perivascular glioma cell displacement of the astrocytic endfeet, astrocyte-released vasoactive molecules (AA, PGE2and K+) can no longer reach the VSMCs to cause alterations in the vessel diameter. Glioma cell PAR1 activation by the artificial ligand, TFLLR, causes increases in glioma cell [Ca2+]i, which activates Ca2+-activated K+channels. Glioma efflux of K+onto VSMCs causes vasoconstriction of the arterioles. Figure 8: Perivascular glioma cells disrupt astrocyte-mediated vascular coupling. The perivascular glioma cell (green) inserts itself between the VSMCs (blue) surrounding the vascular endothelial cells (red), displacing the astrocytic endfeet (purple). Bath application of NE and t-ACPD activates astrocytic G-protein-coupled receptors causing an increase in astrocytic [Ca 2+ ] i . Due to perivascular glioma cell displacement of the astrocytic endfeet, astrocyte-released vasoactive molecules (AA, PGE 2 and K + ) can no longer reach the VSMCs to cause alterations in the vessel diameter. Glioma cell PAR1 activation by the artificial ligand, TFLLR, causes increases in glioma cell [Ca 2+ ] i , which activates Ca 2+ -activated K + channels. Glioma efflux of K + onto VSMCs causes vasoconstriction of the arterioles. Full size image Changes in blood flow are no longer regulated by astrocytes in areas of tumour invasion, which agrees with a reduction of blood flow in glioma patients [53] . Moreover, as contact is lost, astrocytes can no longer transport energy metabolites such as lactate to supply them to neurons [54] . The loss of adequate energy supply may hasten the excitotoxic neuronal demise. Interestingly, a number of other neurological diseases such as Alzheimer’s disease [55] , [56] , hypertension [57] and diabetes [58] have also reported impaired NVC, likely contributing to the complicated pathological processes occurring in each of these diseases. Finally, we show that vessel-associated glioma cells can actively regulate vessel tone. Our data suggest a significant vasoconstriction due to Ca 2+ -activated K + channel-mediated K + release, which we experimentally induced through activation of the PAR1 receptor, which is highly expressed in gliomas [41] . Given that Par1 expression has been reported in other CNS cell types [59] , we complemented this approach by cell type-specific photo-uncaging of Ca 2+ in glioma cells and confirmed a vascular response after artificial Ca 2+ increase in glioma cells. We did not see any response when control vessels were stimulated, suggesting that under our experimental conditions, TFLLR-induced PAR1 activation does not induce the release of vasoactive molecules from astrocytes or the endothelium. Of note, PAR1 receptor activation is likely to occur in human disease [59] . The natural PAR1 ligands are blood-borne thrombin or plasmin [42] , which can enter the brain through the focally breached BBB in areas where gliomas are present. Vasoregulation by K + -release via Ca 2+ -activated K + channels was first shown in cortical astrocytes and depending on [K + ] o , vasodilation or vasoconstriction can occur [9] . Glioma cells highly express Ca 2+ -activated K + channels, including BK and IK channels. Early experiments showed that these channels facilitated invasion and migration [44] , but our studies now suggest a mechanism by which glioma cells use these channels to flux K + to modulate vessel diameter. Glioma-mediated control over vessel diameter may be context specific supporting different aspects of glioma biology. More specifically, invading glioma cells may induce vasoconstriction in an attempt to increase the perivascular space needed to facilitate perivascular invasion. Growing satellite tumours, on the other hand, may benefit from dilated vessels shunting additional blood towards the tumour. In either situation, disrupting this tumour control over blood flow may impair tumour growth or invasion and should be exploited therapeutically in the future. Animals Mice were bred and maintained in a specific pathogen-free barrier facility and all procedures were approved and performed in accordance with guidelines of the Institutional Animal Care and Use Committee (IACUC) of the University of Alabama at Birmingham. Mice were housed in groups of five animals at maximum and subjected to a standard 12 h light/12 h dark cycle. Adult 8–12–week-old C.B.17 scid mice of either sex were used for tumour implantations unless stated otherwise. Immunodeficiency is required to allow growth of tissues derived from a different species, which would otherwise be suppressed by the host’s immune system. Swiss Webster- Aldh1l1-eGFP bacterial artificial chromosome transgenic mice (generated by the GENSAT&#8232;project) were crossed to C.B.17 scid mice and genotyped for the scid Prkdc point mutation as previously described [60] . Mice homozygous for the scid Prkdc mutation and positive for GFP ( Aldh1l1-eGFP-scid ) were maintained as a colony and offspring of either sex was used for experiments. Study design The data contained in the manuscript are not prospective clinical or preclinical trials but instead controlled laboratory experiments pursuing a mechanistic analysis of biological processes in a mouse model of glioma. Hence, we used descriptive statistics for all evaluations. Sample sizes were identical to those used in prior studies of other laboratories, and in each instance, the appropriate reference was listed. Sample sizes were not altered during the study. Surgical procedure Human or mouse glioma cells were implanted into 6–12-week-old immunodeficient C.B.-17 scid or Aldhl1l-eGFP-scid mice of either sex. On the day of surgery, once animals were anesthetized by 2–5% isoflurane, a midline scalp incision was created. A 0.5 mm burr hole was made at 1.0–2.0 mm and 0.5–1.0 mm posterior from the bregma. Gl261-dsRed mouse glioma (1.0–1.5 × 10 5 ), D54-EGFP human glioma cells (1.25-5.0 × 10 5 ), patient-derived xenograft tumours ( GMB14 , GBM22 and GBM39 ; 1.0–1.5 × 10 5 ) or non-malignant glia cells from Aldh1l1-eGFP-scid (0.25–1.0 × 10 5 ) were injected into either one or both hemispheres at 1.0–2.0 mm depth ( z axis at an angle of 35°). Following surgery, intracranial tumours grew for 2–4 weeks. Body weight was monitored periodically and mice showing significant loss of body weight indicating tumour growth were chosen for experiments. Patient-derived xenograft tumour lines Patient xenograft cells were derived from primary brain tumour tissue that was not specifically collected for this project (generous gift by Dr. Yancey Gillespie, Brain Tumour Tissue Core, University of Alabama at Birmingham, Birmingham, AL, USA) and maintained by serial passage in the flank of athymic nude mice, as previously described [22] . In short, tumours were harvested from the flanks after 2–3 weeks. The tissue was chopped into small pieces, waged in phosphate-buffered saline (PBS) and per mouse 200 μl of the solution was injected subcutaneously into the flanks of athymic nude mice to maintain the tumours. The remaining solution was dissociated using GentleMACS Tumour Dissociation Kit (MACS Miltenyl Biotec) and maintained in culture as spheres in Neurobasal-A medium (Invitrogen) supplemented with 10 mg ml −1 of EGF and FGF (Invitrogen), 250 μM ml −1 amphotericin, 50 mg ml −1 gentamycin (Fisher), 260 mM L -glutamine (Invitrogen) and 10 ml B-27 supplement without Vitamin A (Invitrogen). Xenograft cells were maintained as spheres in vitro for 5–7 days before intracranial injections in scid mice. Flank tumours and D54 cells were probed for their VEGF expression profile by western blot analysis. D54 , GBM14 and GBM39 do not show detectable VEGF protein levels, whereas VEGF expression is low in GBM1066 and higher in GBM12 and GBM22 ( Supplementary Fig. 10 ). Glioma preparations for implantation into scid mice Most studies using tumour-bearing mice stereotactically implanted glioma cells derived from D54-MG ( D54 ) glioma cells (WHO IV, glioblastoma multiforme; Dr. D. Bigner, Duke University, Durham, NC) confirmed to exhibit the salient features of the human disease [46] . A stable cell line, D54-eGFP , was generated by transfecting D54-MG cells with pEGFP-N1 (Clonetech) and plasmid insertion was sustained with 0.10 mg ml −1 G418 disulphate salt (Invitrogen). Gl261-dsRed cells were obtained from Frank Winkler (LMU, Munich, Germany). Cells were maintained in Dulbecco’s modified Eagle’s medium/F12 (DMEM/F12) supplemented with 2 mM L -glutamine (Invitrogen) and 7% fetal bovine serum (Aleken Biologicals). Generation of lentiviral plasmids was performed in conjunction with the UAB Neuroscience NINDS Protein Core. To generate a red fluorescing D54 cell line, the pLVX-IRES-tdTomato vector was used. To prepare the lentivirus, pLVK-IRES-tdTomato vectors together with helper plasmids (pPLP1, pPLP2 and pVSVg) were transfected into 293FT cells using Polyfect reagent (Qiagen) per the manufacturer’s recommendations. Seventy-two hours post infection, virus-containing media was collected and stored at −80 °C until utilization. To stably transduce lentiviral vectors into D54 glioma cells, virus-containing supernatant and 3 μg ml −1 Polybrene was added to glioma cells plated 48 h prior to transduction. Twenty-four hours later, the virus-containing medium was exchanged for fresh media and allowed to proliferate for a minimum of 72 h. Following this, a clonal population of TdTomato-expressing D54 cells was selected for the experiments. To generate D54-GCaMP3 cell line, pN1-GCaMP3 (Addgene) was cotransfected using the Cell Line Nucleofector Kit T (Amaxa). D54 cells were plated 48 h prior to transfection to achieve 70–80% confluency. On the day of transfection, the cells were collected and 2 × 10 6 cells were mixed with 3 μg of plasmid DNA in 100 μl of the transfection reagent and electroporated via the Amaxa Nucleofector (Amaxa) using programme T-27. Following electroporation, cell suspension was transferred to six-well cell culture plate (BD Biosciences) with 7% serum-containing media (DMEM/F12) and the media was exchanged the following day. A clonal population of D54-GCaMP3-GFP cells was selected for the experiments. For laser uncaging of Ca 2+ in glioma cells, a D54 clone was used that expressed TdTomato in addition to GCaMP3-GFP. All glioma cells were grown at 37 °C and 90% O 2 /10% CO 2 humidified environment. Glial cell culture obtained from Aldh1l1-eGFP mice The forebrain from 4–7 postnatal Aldh1l1-eGFP-scid mice (2–5 days old) was dissected and mechanically dissociated in Hanks’ buffered saline solution containing 10 mM HEPES. After washing in DMEM medium supplemented with 10% fetal calf serum, 10 mM HEPES and penicillin/ streptomycin, a single-cell suspension was plated into 3 T75 flasks), and the medium was changed every other day. Glial cells were used for intracranial implantations after reaching confluence. Drugs and solutions All chemicals were obtained from Sigma-Aldrich unless otherwise specified. 9,11-dideoxy-9α,11α-methanoepoxy prostaglandin F2α (U46619) and prostaglandin E 2 (PGE 2 ) were obtained from Cayman Chemical and diluted with DMSO, (±)-1-aminocyclopentane- trans -1,3-dicarboxylic acid (t-ACPD), paxilline and Tram-34 were obtained from Tocris Bioscience. Immunohistochemistry Tumour-implanted animals were perfused with PBS followed by 4% paraformaldehyde (PFA) in PBS. Coronal slices (50–100 μm) were sectioned at the vibratome and blocked for 30 min in blocking solution (10% goat serum, 0.5% Triton X in PBS) at room temperature. Any slices stained with antibodies raised in mice were incubated with goat anti-mouse F(ab′) 2 fragment affinity-purified antibody (Jackson Immunoresearch; 1:20) overnight at 4 °C prior to the antibody staining. Slices were then washed in PBS and incubated in primary antibodies, diluted in the blocking solution overnight at 4 °C. Primary antibodies used included mouse Cy3 alpha smooth muscle actin (Sigma-Aldrich; Cat. #C6198; 1:2,000), rabbit aquaporin-4 (Sigma-Aldrich; Cat. #A5971; 1:400), mouse Human Nuclei (Millipore; Cat. #MAB1281 and MAB1281B; 1:100), and ratCD31 (BD Biosciences; Cat. #550274; 1:150). Slices were again washed in PBS and stained with secondary antibodies for 1 h at room temperature. Secondary antibodies used included goat anti-rat Alexa Fluor 647, goat anti-rabbit Cy3, goat anti-rabbit Alexa Fluor 647 and goat anti-mouse Cy3. For antibodies imaged using the 405 nm diode laser, the TSA Plus Coumarin System (Perkin-Elmer) was used per the manufacturer’s instructions. Slices stained with rabbit zonula occludens-1 (ZO-1) (Invitrogen; Cat. #402300) and rabbit claudin-5 (Novus Biologicals; Cat. #NB100-91713) underwent pepsin antigen retrieval (100 mg pepsin in 10 mM hydrochloric acid) for 20 min at 37 °C. Slices were then washed twice with PBST (PBS with 150 μl l −1 Tween-20), incubated in 3% H 2 O 2 for 10 min, and then washed three times with PBS before incubating with primary antibody overnight for a minimum of 48 h at 4 °C. Slices stained with Alexa Fluor 633 hydrazide dye (Invitrogen) were incubated in a 20 μM solution of the dye diluted in PBS for 2 min. Slices were washed with PBS and mounted on glass slides with AquaPolymount (Polysciences). Images were acquired using the Olympus Fluoview FV1000 laser scanning microscope (Olympus) equipped with four diode lasers (405, 473, 559, 635 nm) using a UPLFLN-40X air objective (Olympus). Experiments were successfully repeated; limitations in repeatability of immunohistochemistry or the described results were not encountered. However, tumour sizes and number of migrating tumour cells were variable. Quantification of vessel areas covered by zona occludens-1-positive TJs was done using Fiji/ImageJ. Confocal images of areas with vessels co-opted by D54 glioma cells and neighbouring areas free of tumour were taken. Binary images of 5 μm stacks were created and the area of CD31-positive vessels and ZO-1 was determined. For vessels co-opted by glioma cells, only the vessel area covered by glioma cells was taken into account. To account for variability in the staining from animal to animal, values from glioma images were directly compared with the values of the glioma-free neighbouring region in the same brain section. Western blot Tumour tissue was lysed in RIPA buffer and homogenized using a dounce tissue grinder (Wheaton). After sonication, homogenates were centrifuged for 5 min at 12,000 g at 4 °C. Protein quantification was performed on the supernatant using a BCA protein assay kit (Thermo Scientific). Laemmli-SDS sample buffer, containing 600 mM β -mercaptoethanol, was added to the protein samples before incubating them at 95 °C for 10 min. A quantity of 15 μg of protein was loaded into each lane of a 4–15% gradient precast acrylamide SDS–PAGE gel (Bio-Rad). Samples were separated at 100–200 V. Protein was transferred onto 0.45 μm PVDF transfer membranes (Thermo Scientific, #88518) in Mini Trans-Blot Electrophoretic Transfer Cells (Bio-Rad) at 100 V for 1 h. Membranes were blocked in Tris buffered saline with Tween (TBST) (0.1% Tween-20 in TBS) containing 10% non-fat dried milk for 30 min at room temperature or at 4 °C overnight. Blots were incubated in primary antibody solution (mouse anti-VEGF, Sigma V4758, 2 μg ml −1 ) (TBST, 10% goat serum and antibody) at 4 °C overnight. Blots were washed in TBST 3 × for 10 min and incubated in secondary anti-rabbit, anti-mouse or anti-sheep horseradish peroxidase-conjugated antibody 1:1,500 (Santa Cruz) for 1 h at room temperature. Membranes were washed in TBST 3 × for 10 min and developed using a luminol (Santa Cruz) chemiluminescence kit, and chemiluminescence was detected using a 4000MM Kodak imaging station and Kodak molecular imaging software v.4.0.4. In vivo 2-photon imaging through a cranial window Animals were anesthetized with 2–5% isoflurane. The hair and skin of the skull were removed. A metal bar was secured to the skull behind the lambda by dental cement. Removal of the skull anterior to the lambda and posterior to the bregma was performed on one hemisphere. Animals were injected into the tail vein with 200 μl of 5 mg ml −1 70,000 MW tetramethylrhodamine-dextran (Invitrogen) with a 28 gauge, 0.5 inch long needle (BD Biosciences). Animals were placed on a custom-built apparatus with a heating pad and the metal bar was secured to immobilize the animal’s skull. Arteries and arterioles were identified by their size (<7 μm) and direction of blood flow or by retroorbitally administered Alexa Fluor 633 hydrazide (Invitrogen). Using a multiphoton laser scanning fluorescence microscope (Prairie Technologies) equipped with a X40/0.8 N.A. W water-immersion objective (Olympus) Z stacks of perivascular glioma cells were acquired. Channels were unmixed using ImageJ software and projection images created using Imaris x64 7.5.2 Software (Bitplane Scientific Software). Electron microscopy Tumour-implanted animals were perfused with PBS followed by a fixation solution of 2.5% glutaraldehyde, 4% PFA in 0.1 M sodium cacodylate (Caco) buffer, pH 7.4. After fixation, the brain was removed and sectioned into 100–500 μM slices. Under a fluorescent dissection microscope, tissue punches were taken to capture tumour and non-tumour areas. Punches were placed in fixation solution overnight at 4 °C. Samples were washed two times for 15 min in 0.1 M Caco buffer, pH 7.4 and then immersed in 1% osmium diluted in 0.1 M Caco buffer, pH 7.4 for 50 min at room temperature on a rotator in the dark. Samples were then washed four times in 0.2 M Caco buffer, pH 7.4. Samples were dehydrated in 50, 80 and 95% acetone for 5 min each. Four washes in 100% acetone for 15 min were performed. Samples were equilibrated for embedding in a solution containing equal parts of 100% acetone and Epon 812 with accelerator on a rotator overnight at room temperature. Samples were embedded in 100% Epon 812 with the accelerator at 60–70 °C overnight. Ultrathin sections were cut and imaged on a Tecnai T12 120 kV transmission electron microscope (FEI). BBB permeability assays Tumour-implanted animals were injected with 200 μl of the tracers via tail vein. These tracers were allowed to circulate for 2–3 h before animals were deeply anesthetized and perfused with PBS followed by 4% PFA. Concentration of used tracers was as follows: 2% Evan’s blue (Sigma) in saline, 1 mg ml −1 bovine serum albumin conjugated to Alexa Fluor-555 (Invitrogen) in saline and 500 μg per animal lysine-fixable cadaverine conjugated to Alexa Fluor-555 (Invitrogen) in saline. After adequate fixation, 50–100 μm coronal slices were cut and immunohistochemistry was performed as described above. For the in vivo tracer injection experiments, 100 μl of 12.5 mg ml −1 10,000 MW Cascade Blue (Invitrogen) and Alexa Fluor 633 hydrazide dye (0.2 mg ml −1 ) was retroorbitally injected. These animals were anesthetized with 2–5% isoflurane and placed on a custom-built apparatus with a heating pad and the metal bar was secured to immobilize the animal’s skull. Images were acquired using a 4-detector Olympus FV-1000MPE multiphoton laser scanning microscope with a Coherent Chameleon Vision II Ti:Sapphire laser (Olympus) with a XLPN 25X/1.05 N.A. water-immersion objective to visualize four different dyes. Channels were unmixed using Olympus Fluoview Software Version 3.1b. Projection images were created using ImageJ software. Acute brain slice drug application experiments Animals were killed and brains were placed in ice-cold artificial cerebrospinal fluid (cutting ACSF) bath solution (135 mM N -methyl- D -glucamine, 1.5 mM KCl, 3.5 mM MgSO 4 , 0.5 mM CaCl 2 , 1.5 mM KH 2 PO 4 , 23 mM choline bicarbonate, 25 mM D -glucose and 0.4 mM ascorbic acid bubbled with 95% O 2 /5% CO 2 to maintain pH at 7.4). A quantity of 200 μm coronal slices were sectioned and allowed to recover for 45 min to 1 h at 28 °C in recording ACSF (125 mM NaCl, 3.0 mM KCl, 1.25 mM NaH 2 PO 4 , 25 mM NaHCO 3 , 25 mM D -glucose, 2.0 mM CaCl 2 , 2.0 mM MgSO 4 ) bubbled with 95% O 2 /5% CO 2 to maintain pH at 7.4. When specified, vessels were preconstricted in 125 nM U46619 for 20 min in recording ACSF bubbled with 95% O 2 /5% CO 2 at 37 °C. For experiments at ‘low oxygen’ concentrations, slices were transferred to recording ACSF bubbled with 20% O 2 /5% CO 2 for a minimum of 20 min before the onset of the experiment. Acute brain slices were transferred to a Leica DM LFSA upright DIC-IR fluorescence microscope using a Zeiss Hm digital camera at × 1000 magnification (Leica Microscopy). Slices were continually perfused with recording ACSF heated to 33 °C and bubbled with ‘high oxygen’ conditions (95% O 2 /5% CO 2 ) or ‘low oxygen’ conditions (20% O 2 /5% CO 2 ). Timelapse images of vessels were acquired using Axiovision 4.7 software (Carl Zeiss Microscopy). Vessel diameter was measured as the cross-section of the vessel using ImagePro (Media Cybernetics) or ImageJ software (NIH Image, NIH). Acute brain slice calcium uncaging experiments After obtaining slices as described above, slices were allowed to recover for 1 h in ACSF bubbled with 95% O2/5% CO2 at room temperature to maintain pH at 7.4). Slices were loaded with 40 μM Alexa Fluor 633 Hydrazide (Invitrogen), 10 μM Fluo-4 acetoxymethyl ester AM (Invitrogen) Ca 2+ indicator, and 10 μM DMNPE-4 caged Ca 2+ [36] in ACSF containing 0.02% pluronic acid for 60 min at room temperature. Slices were then transferred to regular ACSF to allow for stabilization before recording. Alexa Fluor 633 Hydrazide and Fluo-4 AM fluorescence was detected by laser scanning confocal microscopy using an Olympus FV1000 and a 60 × /1.1 NA water-immersion objective (Olympus). Single plane confocal images of 800 × 800 or 640 × 640 pixels were obtained approximately every 2 s. Ca 2+ uncaging was achieved using a 405 nM laser in region of interest tornado scanning mode at 40% power for 800 ms that was directed at astrocytic endfeet associated with arterioles identified by Alexa Fluor 633 Hydrazide dye. Vessel diameter was measured as the cross-section of the vessel using ImageJ software (NIH Image, NIH). Statistical analysis All data obtained was analysed using Origin 6.0 software (Microcal Software). Statistical tests were performed using GraphPad Instat (GraphPad Software Inc,) or GraphPad Prism 6.0; specific tests are stated in the results. All measurements are reported with standard error of mean. The KS normality test was performed for each data group. If normality was not achieved, a Mann–Whitney test was performed instead of the unpaired t -test. The specific test is stated in the results and figure legends. No data/outliers were excluded from the analysis. The number of replicates is reported in the results and figure legends. How to cite this article: Watkins, S. et al. Disruption of astrocyte–vascular coupling and the blood–brain barrier by invading glioma cells. Nat. Commun. 5:4196 doi: 10.1038/ncomms5196 (2014).